Pattern recognition algorithm reveals how birds evolve individual egg pattern signatures Pattern-based identity signatures are commonplace in the animal kingdom, but how they are recognized is poorly understood. Here we develop a computer vision tool for analysing visual patterns, N ATURE P ATTERN M ATCH , which breaks new ground by mimicking visual and cognitive processes known to be involved in recognition tasks. We apply this tool to a long-standing question about the evolution of recognizable signatures. The common cuckoo ( Cuculus canorus ) is a notorious cheat that sneaks its mimetic eggs into nests of other species. Can host birds fight back against cuckoo forgery by evolving highly recognizable signatures? Using N ATURE P ATTERN M ATCH , we show that hosts subjected to the best cuckoo mimicry have evolved the most recognizable egg pattern signatures. Theory predicts that effective pattern signatures should be simultaneously replicable, distinctive and complex. However, our results reveal that recognizable signatures need not incorporate all three of these features. Moreover, different hosts have evolved effective signatures in diverse ways. Recognition of kin, mates, neighbours, rivals and predators is a widespread and critical feature of animal societies. Individual recognition occurs when one organism (the receiver) identifies another (the signaller) based on individually distinctive characteristics or signatures [1] , [2] . Signatures are common in diverse taxa. They can be chemical, like the hydrocarbon signatures used by Formica ants to recognize nest-mates [3] , or auditory, like the vocalizations used by Australian sea lion ( Neophoca cinerea ) mothers and pups to reunite in dense colonies [4] , or visual, like the facial patterns used by Polistes fuscatus paper wasps to recognize individuals in the colony [5] . In birds, egg patterns can be visual signatures of offspring identity, enabling parents to recognize their eggs in a crowded colony [6] or to distinguish their own eggs from those of a brood parasitic cheat [7] . How do signatures evolve to actively promote recognizability? Although many studies have established that receivers can discriminate individuals on the basis of visual signatures, little work has addressed the question of how signallers broadcast specific signature cues to enhance recognizability [2] , [8] , in part because we lack sophisticated tools for quantifying signature information appropriately. Consequently, the evolution of distinctive visual signatures and the mechanisms by which animals interpret them remain poorly understood. Parasite–host systems provide a compelling opportunity to investigate the evolution of recognizable signatures. Parasites commonly mimic host appearance, sound, smell or chemical makeup to exploit hosts, and many hosts escape parasite mimicry by evolving recognizable signatures in response. Cuckoo–host interactions are ideal for examining how hosts might evolve phenotypic signatures that are easy to recognize yet difficult to copy. The interactions between the common cuckoo ( Cuculus canorus ) and its European hosts are now a textbook example of coevolution [9] , [10] . Cuckoo females belong to different genetic races, each of which selectively targets a host species. To sneak their eggs into host nests, many cuckoo host-races have evolved remarkable egg mimicry [11] , [12] , [13] , [14] . Hosts can then defend themselves by evolving better discrimination abilities or by evolving more recognizable egg pattern signatures that facilitate detection of an imposter egg [9] , [15] , [16] . Evidence for enhanced discrimination by hosts comes from many studies demonstrating that host discrimination of foreign eggs is at its most refined in species that are parasitized by common cuckoo host-races with near-perfect egg mimicry [11] , [12] , [13] , [14] . However, evidence for the evolution of recognizable egg pattern signatures by common cuckoo hosts is more mixed [7] . Do hosts of the common cuckoo mark their eggs with recognizable signatures? Theory predicts that effective egg pattern signatures should have three features [17] , [18] , [19] . First, a signature should be replicable (low intraclutch variation). Hosts should evolve less variation in their own clutches because a faithfully repeated signature increases the ease with which the host can spot and reject the parasitic egg [18] , [19] . Second, a signature should be distinct from those of other females (high interclutch variation). Selection should favour hosts whose clutches differ greatly from each other [17] , [18] , [19] , [20] . This makes it challenging for a cuckoo to evolve a close match to all signatures simultaneously. Third, a signature should be difficult to reproduce (high complexity). Hosts should evolve signatures that are too complex for parasites to forge, just as banks deter counterfeiters by creating complex banknotes with increasingly outlandish watermarks [17] , [19] . The general assumption has been that host signatures should evolve to possess these three features (replicability, distinctiveness and complexity) simultaneously. However, comparative studies that have searched for independent correlations between host rejection behaviour (that is, the frequency of rejection of a foreign egg) and these different signature features have yielded equivocal results [18] , [19] , [21] , [22] . This might be because the approach of separately evaluating different signature features oversimplifies the cognitive processes involved in signature recognition. If a signature is highly replicable, perhaps it can be recognizable without being highly distinctive or complex. Furthermore, these previous analyses were based on subjective, human-derived rankings of clutch variation and complexity. Yet the relevant signal receiver here is the host bird faced with the challenge of distinguishing its own eggs from cuckoo forgeries [23] , [24] . Understanding the evolution of recognizable egg signatures therefore involves modelling how a bird brain processes pattern information. Although existing models of avian vision provide many advantages over approaches based on human vision [25] , the available models for assessing colour (for example, photoreceptor sensitivity) and pattern (for example, Fourier analysis) are largely based on early-stage, low-level visual processes and so fall short of capturing higher-order cognitive processes involved in pattern recognition. In this study, we create an advanced computer vision tool for evaluating the recognizability of natural patterns and we apply it specifically to the question of whether hosts of the common cuckoo have evolved eggs with individual pattern signatures. We ask: if recognizable signatures have evolved, what features make them easily detectable? We first use a camera specifically calibrated for bird vision to photograph eggs laid by eight of the common cuckoo’s favourite European hosts. To then quantify egg pattern signatures as the avian brain might process them, we introduce N ATURE P ATTERN M ATCH , a computer vision programme based on object recognition algorithms that detect, describe and compare local features in a visual scene [26] , [27] . These ‘signature’ features are analogous to those used by primates and birds in real object recognition tasks [28] , [29] . For each host species, we then conduct a simulation in which each egg image must be matched to its correct clutch on the basis of its pattern alone, yielding a single measure of signature recognizability. Using this multidisciplinary approach, which combines tools from computational neuroscience, sensory ecology and cognition, we investigate egg pattern signatures in a way that accounts for avian visual neurobiology, thus permitting a new look at the unsolved mystery of whether hosts fight back against common cuckoo mimicry by evolving special egg patterns of their own. Overall, our method represents a new way to examine how animals encode and recognize signature information. Estimating a bird brain’s view of host egg signatures Using the collections of the Natural History Museum (Tring, Hertfordshire, UK), we photographed 689 host eggs from 206 cuckoo-parasitized clutches (each containing host eggs and a cuckoo egg) belonging to eight of the cuckoo’s preferred European hosts ( Fig. 1 ): dunnock ( Prunella modularis ), meadow pipit ( Anthus pratensis ), reed warbler ( Acrocephalus scirpaceus ), garden warbler ( Sylvia borin ), great reed warbler ( Acrocephalus arundinaceus ), brambling ( Fringilla montifringilla ), pied wagtail ( Motacilla alba ) and red-backed shrike ( Lanius collurio ). Although one host, the dunnock, lays immaculate eggs, the remaining host species lay eggs variably covered with pattern markings. To investigate the effects of egg pattern signatures independently of egg background colour, we focused exclusively on egg patterning (or maculation), which includes the speckles, scrolls and markings formed by protoporphyrin pigment on the eggshell’s surface [7] . In birds, luminance (achromatic) vision is processed independently of colour, stems from a set of receptors called double cones and is likely important for tasks related to pattern and texture perception [30] . Therefore, we recalibrated our photographs in terms of bird luminance vision [13] , [30] , providing an estimate of how a bird’s double cones would be stimulated upon seeing an egg ( Figs 1 and 2 ). 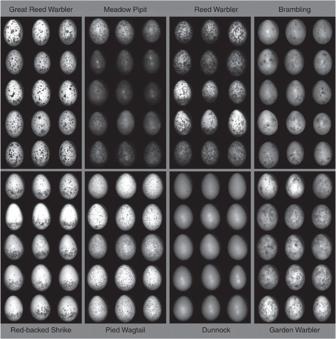Figure 1: Eggs laid by hosts of the brood parasitic common cuckoo. Shown here are eggs laid by eight hosts of the common cuckoo (Cuculus canorus). For each species, eggs from five different clutches are shown, with three representative eggs per clutch. For all hosts in our sample, the median clutch size was either three or four eggs. Each row represents a unique clutch. Egg images were calibrated for avian luminance vision. For clarity, the overall image has been brightened by 20%. Egg images by M.C.S. and copyright NHM. Figure 1: Eggs laid by hosts of the brood parasitic common cuckoo. Shown here are eggs laid by eight hosts of the common cuckoo ( Cuculus canorus ). For each species, eggs from five different clutches are shown, with three representative eggs per clutch. For all hosts in our sample, the median clutch size was either three or four eggs. Each row represents a unique clutch. Egg images were calibrated for avian luminance vision. For clarity, the overall image has been brightened by 20%. Egg images by M.C.S. and copyright NHM. 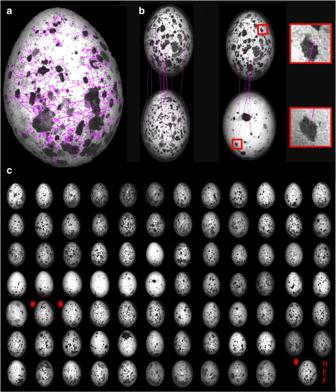Figure 2: Detecting and matching distinctive features of egg patterns laid by hosts of the common cuckoo. Shown here are eggs of the great reed warbler (Acrocephalus arundinaceus). (a) The SIFT algorithm extracts features on a host egg. Each vector, indicated by a magenta arrow, corresponds to a unique SIFT keypoint feature. The length of the vector corresponds to the feature’s dominant scale (or size), and the direction of the vector corresponds to the feature’s dominant orientation. (b) A novel pattern matching algorithm then compares a reference egg to all other eggs in a specified library. Here, the same egg (top row) is compared with two eggs from different clutches. The magenta lines connect those SIFT features in each pair of images that are considered matches by our algorithm. The first pair of eggs (left column) has a greater number of matching features than those in the second pair (right column), and indeed the eggs in the first pair (left) originated from the same clutch while those in the second pair (right) did not. It is possible for eggs from different clutches to have occasional features that are similar (see red boxes), but—among hosts with recognizable signatures—these spurious ‘matches’ will be small in number compared with the number of matching features shared by eggs laid by the same female. (c) Eggs from 26 clutches laid by different great reed warblers. Using NATUREPATTERNMATCH, the reference egg (lower right) was correctly matched—on the basis of the egg pattern alone—to its target clutch (red asterisks) on the first attempt, demonstrating that this particular female has a highly recognizable pattern signature. Overall, great reed warblers had the fourth (of eight) most recognizable pattern signatures among common cuckoo hosts. Eggs are not shown to scale. Egg images by M.C.S. and copyright NHM. Full size image Figure 2: Detecting and matching distinctive features of egg patterns laid by hosts of the common cuckoo. Shown here are eggs of the great reed warbler ( Acrocephalus arundinaceus ). ( a ) The SIFT algorithm extracts features on a host egg. Each vector, indicated by a magenta arrow, corresponds to a unique SIFT keypoint feature. The length of the vector corresponds to the feature’s dominant scale (or size), and the direction of the vector corresponds to the feature’s dominant orientation. ( b ) A novel pattern matching algorithm then compares a reference egg to all other eggs in a specified library. Here, the same egg (top row) is compared with two eggs from different clutches. The magenta lines connect those SIFT features in each pair of images that are considered matches by our algorithm. The first pair of eggs (left column) has a greater number of matching features than those in the second pair (right column), and indeed the eggs in the first pair (left) originated from the same clutch while those in the second pair (right) did not. It is possible for eggs from different clutches to have occasional features that are similar (see red boxes), but—among hosts with recognizable signatures—these spurious ‘matches’ will be small in number compared with the number of matching features shared by eggs laid by the same female. ( c ) Eggs from 26 clutches laid by different great reed warblers. Using N ATURE P ATTERN M ATCH , the reference egg (lower right) was correctly matched—on the basis of the egg pattern alone—to its target clutch (red asterisks) on the first attempt, demonstrating that this particular female has a highly recognizable pattern signature. Overall, great reed warblers had the fourth (of eight) most recognizable pattern signatures among common cuckoo hosts. Eggs are not shown to scale. Egg images by M.C.S. and copyright NHM. Full size image To investigate how the egg pattern might then be processed by the avian brain, we created a computer programme, N ATURE P ATTERN M ATCH , which uses the Scale-Invariant Feature Transform (SIFT) [26] , [27] to detect the important features of each egg pattern (for technical details, see Supplementary Note 1 ). In the same way that a topographer might identify the most interesting features of a landscape, SIFT locates and extracts keypoint features associated with individual markings of an egg’s pattern ( Fig. 2a ). SIFT features are extracted in a way that mimics the response of neurons in the primate inferior temporal cortex [26] , [29] , which plays a crucial role in object recognition. The extracted features correlate with parts of a visual scene to which primates are most likely to pay attention [31] . Although birds do not have structures homologous to those in the ventral stream of the primate visual cortex, the avian tectofugal pathway—which plays a dominant role in visual discrimination tasks—is believed to operate in a similar way, with recent work supporting the view that the general processes involved in object recognition are widely conserved in vertebrates [28] . In primates and birds, visual processing occurs in different regions of the brain, with different features extracted and represented at various stages of the visual pathway [28] , [32] , [33] . In the early stages, simple local features, such as lines, corners and edges, are encoded. In later stages, neurons encode features with intermediate complexity, such as shapes or markings that are largely invariant to transformation and rescaling; SIFT extracts and analyses these features of intermediate complexity [26] , [29] . Intermediate features likely play a specific and important role in object classification in primates [33] , and recent evidence suggests that birds too make use of these features in object recognition tasks [28] , [34] . Thus, SIFT evaluates patterns in a way that is neurobiologically plausible, not just for primates but also for birds, providing a sophisticated method for investigating patterns as they may actually be perceived by the avian brain. However, many aspects of avian pattern recognition remain poorly understood [28] , so our model provides a roughly analogous representation rather than a complete description of the cognitive processes involved in avian pattern perception. Discovering which biologically inspired models of object recognition best approach the capabilities of real primate and avian visual systems is an important goal for the future [35] . Following extraction of SIFT features, N ATURE P ATTERN M ATCH uses these features to compare a given egg pattern to all other eggs laid by females of the same species and computes an overall similarity score based on the relative number of descriptors that can be matched between each pair of images ( Fig. 2b ). For each host species, we were thus able to calculate how closely, on average, a given egg matched its own clutch ( Fig. 2c ). Our measure of signature recognizability is the likelihood that an egg will be correctly matched to its own clutch in the first three attempts. In addition to quantifying overall signature recognizability, we conducted cluster analyses on egg features to derive measures of intraclutch variation (replicability) and interclutch variation (distinctiveness) for each host species. To test the idea that recognizable signatures should also be complex, we first calculated a measure of visual density based on the average number of SIFT features per egg, which we subsequently log-transformed. As feature density is a simple proxy for complexity and does not contain spatial information, we also calculated the spatial dispersion of egg patterns, which is based on the average spacing between egg pattern features. Hosts have evolved recognizable egg signatures If hosts and their respective cuckoo host-races are locked in different stages of a coevolutionary arms race [9] , we would expect those hosts subjected to the best cuckoo egg mimicry to have evolved the most recognizable egg signatures in response ( Supplementary Fig. 1 ). We compared host signature recognizability to previously established measures of cuckoo egg pattern mimicry [13] and found that hosts have indeed evolved recognizable signatures as a defence against cuckoo parasitism ( Fig. 3a ; weighted linear regression: F 1,7 =18.84, P =0.005, R 2 =0.76, n =8). The brambling, which lays a light blue egg spotted with small, unevenly spaced red-brown blotches, has evolved the most recognizable signature in response to apparently excellent pattern mimicry by its respective cuckoo host-race. In contrast, the dunnock, which lays an immaculate blue egg, has no egg pattern signature at all. The dunnock appears to be at an early stage of the arms race and has not yet evolved rejection defences [11] . Consequently, the cuckoo host-race that targets dunnocks has not been under selection for mimetic eggs, and dunnocks have not been exposed to selection for signatures to escape mimicry. 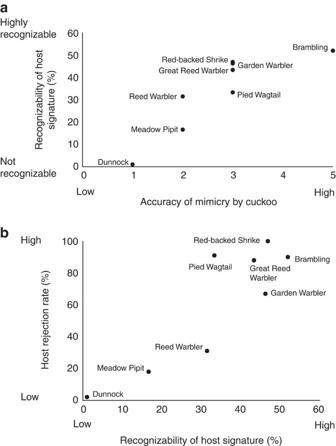Figure 3: Recognizability of host eggs is correlated with cuckoo egg mimicry and predicts host rejection behaviour. (a) The relationship between the degree of cuckoo pattern mimicry (data taken from the study by Stoddard and Stevens13) and the recognizability of the host pattern signature. Weighted linear regression,P=0.005. (b) The relationship between the recognizability of the host egg signature and the frequency with which hosts reject non-mimetic eggs. Rejection rates are from the study by Avilés and Garamszegi36. Weighted linear regression,P=0.004. These results indicate that hosts of the common cuckoo have evolved modified egg patterns in response to cuckoo mimicry (a), leading to recognizable pattern signatures that facilitate rejection of parasitic eggs (b). Recognizability of the host signature is measured as the likelihood that a host egg will be correctly identified to its own clutch (see text for details). Figure 3: Recognizability of host eggs is correlated with cuckoo egg mimicry and predicts host rejection behaviour. ( a ) The relationship between the degree of cuckoo pattern mimicry (data taken from the study by Stoddard and Stevens [13] ) and the recognizability of the host pattern signature. Weighted linear regression, P =0.005. ( b ) The relationship between the recognizability of the host egg signature and the frequency with which hosts reject non-mimetic eggs. Rejection rates are from the study by Avilés and Garamszegi [36] . Weighted linear regression, P =0.004. These results indicate that hosts of the common cuckoo have evolved modified egg patterns in response to cuckoo mimicry ( a ), leading to recognizable pattern signatures that facilitate rejection of parasitic eggs ( b ). Recognizability of the host signature is measured as the likelihood that a host egg will be correctly identified to its own clutch (see text for details). Full size image Once cuckoo mimicry has selected for more recognizable host signatures, do host signatures influence the ease with which hosts identify and reject foreign eggs ( Supplementary Fig. 1 )? We compared host signature recognizability to previously established measures of host rejection behaviour [36] and found that hosts with the most recognizable pattern signatures are the best at rejecting non-mimetic foreign eggs ( Fig. 3b ; weighted linear regression: F 1,7 =20.89, P =0.004, R 2 =0.78, n =8). Note that experimental rates of rejection of non-mimetic eggs are considered to be a proxy for the discrimination abilities of hosts [22] . Characteristics of a recognizable signature A long-standing general prediction of the signature hypothesis is that hosts should evolve clutches with low intraclutch variation (high replicability) and high interclutch variation (high distinctiveness) [17] , [18] , [19] . Surprisingly, we did not find that low intraclutch variation is correlated with high interclutch variation. Instead, the relationship between intraclutch and interclutch variation can be described by a quadratic curve, with intermediate values of intraclutch variation corresponding to the highest values of interclutch variation ( F 2,203 =807.18, P <0.001, R 2 =0.89, n =8). The quadratic relationship was still significant when the dunnock, which lays immaculate eggs, was omitted from the analysis. This relationship suggests that host patterns, in general, can be characterized by low intraclutch variation or high interclutch variation, but not both at the same time. Instead, patterns with moderate intraclutch variation typically have the highest interclutch variation, while patterns with low or high intraclutch variation typically have low interclutch variation. A second general prediction of the signature hypothesis is that hosts should evolve egg patterns that are complex and therefore difficult to forge. Do hosts with highly recognizable signatures have egg patterns that are visually complex? We compared the degree of recognizability to our measure of visual density, which is the average number of SIFT features per egg (log-transformed). Some species, like the great reed warbler and the pied wagtail, lay eggs densely covered with features (high visual density), while others like the brambling and dunnock lay eggs with few or no features, respectively (low visual density). Surprisingly, the most recognizable egg pattern signatures are not those with the highest visual density ( Figs 4a and 5 ). The relationship between pattern recognizability and visual density was best described by a quadratic model (F 2,203 =2,965.67, P <0.001, R 2 =0.97, n =8), which remained significant even when the dunnock was removed from the analysis. Therefore, the most recognizable signatures are those with an intermediate number of features. If there are too few features or too many features, recognizability declines. In this sense, it appears that a high density of features can compromise overall recognizability. One possible explanation is that as visual density increases beyond a certain threshold, the eggshell becomes so covered in markings that there are fewer ways for its pattern to stand out. This concept—that increased complexity can actually result in reduced accuracy of a predictive model—is fundamental to information theory and machine learning [37] , yet relatively new to biological systems. 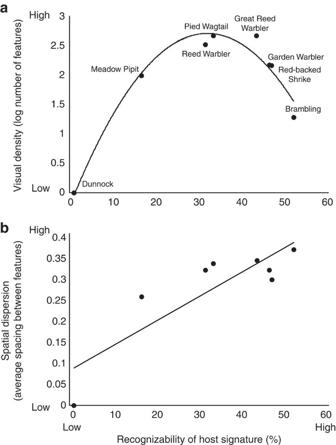Figure 4: Recognizability of host egg patterns is related to visual density and spatial dispersion. (a) The most recognizable signatures (brambling, red-backed shrike and garden warbler) tend to have intermediate levels of visual density. Egg signatures with the highest visual density (reed warbler, pied wagtail and great reed warbler) are less recognizable. Quadratic model,P<0.001. (b) Signature recognizability is positively correlated with the degree of spatial dispersion in egg patterns. Weighted linear regression,P=0.007. Spatial dispersion is high in egg patterns exhibiting a high degree of spacing between distinctive features, such as in the brambling. Spatial dispersion may be a more reliable indicator of signature information content than visual density (a). Figure 4: Recognizability of host egg patterns is related to visual density and spatial dispersion. ( a ) The most recognizable signatures (brambling, red-backed shrike and garden warbler) tend to have intermediate levels of visual density. Egg signatures with the highest visual density (reed warbler, pied wagtail and great reed warbler) are less recognizable. Quadratic model, P <0.001. ( b ) Signature recognizability is positively correlated with the degree of spatial dispersion in egg patterns. Weighted linear regression, P =0.007. Spatial dispersion is high in egg patterns exhibiting a high degree of spacing between distinctive features, such as in the brambling. Spatial dispersion may be a more reliable indicator of signature information content than visual density ( a ). 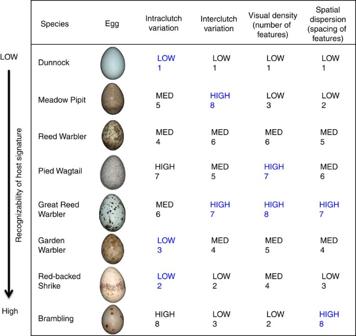Figure 5: Diversity of host egg pattern signatures. To achieve recognizable signatures, hosts have evolved patterns with different combinations of intraclutch variation (replicability), interclutch variation (distinctiveness), visual density and spatial dispersion. However, the most recognizable signatures are not simultaneously replicable, distinctive and visually complex. ‘High, ‘Medium’ and ‘Low’ refer to the rank relationships between host species, which are also shown numerically. Rankings are from 1 (lowest) to 8 (highest). For intraclutch variation, a rank of 1 represents high replicability and a rank of 8 represents low replicability. For interclutch variation, a rank of 1 represents low distinctiveness and a rank of 8 represents high distinctiveness. For visual density, a rank of 1 represents low visual density and a rank of 8 represents high visual density. For spatial dispersion, a rank of 1 represents low spatial dispersion (closely spaced features) and a rank of 8 represents high spatial dispersion (widely spaced features). Features believed to enhance recognizability are highlighted in blue. Egg images by M.C.S. and copyright NHM. Full size image Figure 5: Diversity of host egg pattern signatures. To achieve recognizable signatures, hosts have evolved patterns with different combinations of intraclutch variation (replicability), interclutch variation (distinctiveness), visual density and spatial dispersion. However, the most recognizable signatures are not simultaneously replicable, distinctive and visually complex. ‘High, ‘Medium’ and ‘Low’ refer to the rank relationships between host species, which are also shown numerically. Rankings are from 1 (lowest) to 8 (highest). For intraclutch variation, a rank of 1 represents high replicability and a rank of 8 represents low replicability. For interclutch variation, a rank of 1 represents low distinctiveness and a rank of 8 represents high distinctiveness. For visual density, a rank of 1 represents low visual density and a rank of 8 represents high visual density. For spatial dispersion, a rank of 1 represents low spatial dispersion (closely spaced features) and a rank of 8 represents high spatial dispersion (widely spaced features). Features believed to enhance recognizability are highlighted in blue. Egg images by M.C.S. and copyright NHM. Full size image Perhaps the spacing of features, rather than the absolute number of features, is a more important predictor of signature recognizability: maybe spatially distinct landmarks are more easily recognized than a dense constellation of features. To test this, we devised a measure of spatial dispersion, such that patterns with large distances between features have high spatial dispersion and those with small distances between features have low spatial dispersion. Note that spatial dispersion is not necessarily inversely related to our measure of visual density (the number of features) since some eggs, like those of the great reed warbler, have many features overall but retain a high level of spacing between them. Brambling eggs, with their large but sparse blotches, have the highest spatial dispersion. Meadow pipit eggs, which have small but dense speckles, have the lowest spatial dispersion, with the exception of immaculate dunnock eggs. Do the most recognizable signatures have the greatest degree of spatial dispersion? We found a strong positive correlation between pattern recognizability and spatial dispersion ( Fig. 4b ; weighted linear regression: F 1,7 =16.20, P =0.007, R 2 =0.73, n =8). This result was still significant when the dunnock was omitted from the analysis. Overall, these results suggest that the most recognizable pattern signatures tend to have higher spatial dispersion but not necessarily a higher density of features. There appears to be a cost associated with having a visually dense signature, contrary to the original prediction of the signature hypothesis that the optimal signature should have a high degree of visual complexity. Rather, the ideal signature should have an intermediate degree of visual density with at least some features that are spatially distinct ( Fig. 5 ). We have used two straightforward measures, feature density and spatial dispersion, as proxies for visual complexity. Although these measures do not capture all aspects of pattern complexity, their interpretation is straightforward and they do have clear effects on the recognizability of patterns. Other aspects of pattern variation (such as marking size, variation in marking size and variation in spacing) may further contribute to visual complexity: we measured these characteristics for all eggs and discuss trends in Supplementary Note 1 . Is it possible to combine these measures into one unified measure of complexity? Although there are several proposed measures of visual complexity, there is no clear agreement on their appropriateness and applicability, though this is an area of active research [38] . Some of the difficulties may stem from the fact that complexity is challenging to define: are the small, dense markings on pied wagtail eggs more complex than the irregular blotches of the brambling egg, or vice versa? Since either alternative is possible, we devised measures that capture both potential aspects of complexity: density and spacing. In the future, it will be critical to determine how visual complexity relates to true mechanistic complexity ( Supplementary Table 1 ). Our assumption has been that complex egg patterns are desirable in hosts because they are difficult for cuckoos to forge. However, without detailed physiological study of the cuckoo oviduct, it is not yet clear that this is the case. Here we develop a novel pattern recognition tool, N ATURE P ATTERN M ATCH , which is inspired by neurobiology and can be used to detect, recognize and compare a broad range of natural patterns in a wide diversity of species. In future work, N ATURE P ATTERN M ATCH can be employed in investigations of recognition and learning, visual communication and camouflage, and pattern heritability. Here it has yielded new insights into the evolution of identity signatures by hosts of avian brood parasites. Our analysis reveals remarkable sophistication in the evolution of egg signatures by hosts of the common cuckoo. Many hosts have indeed evolved individual, highly recognizable egg pattern signatures as a defence against cuckoo egg mimicry ( Fig. 3a ), and host signatures influence the ease with which hosts identify and reject foreign eggs ( Fig. 3b ). Overall, egg identity signals may be a more potent and widespread defence against parasitic forgeries than previously realized because the phenomenon is more cryptic than is readily apparent to the human eye. Which signature strategies have different hosts pursued? The four host species with the most recognizable pattern signatures—brambling, red-backed shrike, garden warbler and great reed warbler—have evolved successful signatures in different ways ( Fig. 5 ). Brambling eggs have high intraclutch variation, low interclutch variation and low visual density, in exact opposition to the prediction of the signature hypothesis. Yet the brambling has evolved the most recognizable signature. How? Brambling eggs have the highest degree of spatial dispersion, which may make its sparse features more easily recognized, in the same way that distinctive landmarks stand out in a landscape. The red-backed shrike and garden warbler, by contrast, have evolved egg patterns that are not highly spatially dispersed—nor are they visually dense or highly distinctive. However, their egg patterns have very low intraclutch variation (high replicability), which likely contributes to their high degree of recognizability. The great reed warbler has evolved eggs with only a modest degree of intraclutch variation but a high degree of interclutch variation (high distinctiveness); its pattern also has high visual density and high spatial dispersion. With high distinctiveness, high visual density and high spatial dispersion, we might expect the great reed warbler to have eggs that are even more recognizable. However, the great reed warbler egg pattern’s high visual density (highest of all the hosts) may actually serve to reduce its recognizability if too many features make the scene noisy. It is interesting to note that the highly effective pattern signatures of the brambling, red-backed shrike and garden warbler are characterized by only low-to-moderate visual density. Perhaps recognition based on template learning, believed to be the rule among highly discriminating hosts like these [39] , works best if the signature is not overly complex or dense. Future experiments could test this idea by manipulating the visual complexity of egg pattern signatures and determining how this affects recognition and rejection behaviour in the field. At the other end of the spectrum, pied wagtails, reed warblers and meadow pipits have not evolved highly recognizable egg signatures ( Fig. 5 ). Pied wagtail eggs have high visual density in addition to high intraclutch variation, intermediate interclutch variation and intermediate spatial dispersion, none of which is expected to enhance recognizability. Reed warbler eggs are similar, with intermediate measures of intraclutch variation, interclutch variation, visual density and spatial dispersion. Meadow pipit eggs possess the highest interclutch variation, which in theory should boost recognizability, but perhaps the high distinctiveness of the egg pattern is insufficient to compensate for its modest replicability, low visual density and low spatial dispersion. Finally, the immaculate blue eggs of the dunnock are highly replicable but wholly indistinctive, not visually dense and completely lacking in spatial information, rendering them unrecognizable. Although our study confirms the evolution of recognizable signatures in several host species, our findings challenge two central features of the traditional signature hypothesis. First, contrary to classic assumptions about signature evolution, there are several ways to evolve a recognizable signature. Previous theoretical work suggested that all hosts will eventually evolve egg polymorphisms (high interclutch variation) [40] . However, our results indicate that this is just one possible outcome of signature evolution: alternatively, hosts can evolve highly effective signatures that are replicable or difficult to forge without necessarily being polymorphic. These results highlight the importance of investigating identity signals across multiple species: not all identity signals will conform to the same criteria. Second, no egg patterns are simultaneously replicable, distinctive and complex. Instead, hosts have elaborated their signatures in different ways, optimizing some security features instead of others ( Fig. 5 ). Moreover, the most effective egg pattern signatures are not those with the highest visual density of features. The three hosts with the most recognizable pattern signatures (brambling, red-backed shrike and garden warbler) do not have signatures with the highest visual density, perhaps because this degree of complexity makes signatures less recognizable ( Fig. 4a ). Instead, the ideal pattern may be one that is complex enough to be distinctive but not so complex that meaningful information is lost. In general, the precise genetic and physical mechanisms underlying pigment pattern formation on eggs remain unclear. Discovering how genetic and physical processes affect replicability, distinctiveness, density and spatial dispersion of egg patterns will be key to understanding possible constraints on the evolution of recognizable signatures by hosts ( Supplementary Table 1 ). As phylogenetic constraints may also influence the evolution of certain egg patterns [7] , it will be important ultimately to investigate the extent of egg pattern replicability, distinctiveness and complexity in different avian lineages. Bird eggs are under diverse selection pressures [7] , [41] and this may additionally influence the type of signature that eventually evolves. Is there a cost to having a complex signature? Our findings demonstrate that the ‘banknote’ analogy [9] , [19] , which suggests that complex signatures are always desirable, does not always apply. In fact, increased pattern complexity—at least in terms of the absolute number of features (density)—comes at a cost to overall recognizability. If host egg patterns are to retain a high degree of recognizability, then the ideal pattern is one that is visually dense enough to be informative but not so dense that it becomes unrecognizable due to high entropy. This idea is well established in computer science, in which trade-offs between complexity and information form the basis for algorithmic information theory [37] . We acknowledge that there are many ways to characterize visual complexity, and several detailed studies have been devoted to this topic [38] . In this study, we aimed to identify two important and quantifiable aspects of pattern variation (feature density and spatial dispersion) that appear to influence a pattern’s overall recognizability. In future tests of the signature hypothesis for egg patterns, it will be crucial to define complexity clearly and to explore alternative metrics for capturing complex visual patterns. Furthermore, linking visual complexity to the mechanisms of pattern formation in the shell gland (that is, production of spots versus scrolls or squiggles) may clarify whether patterns that appear to be complex are in fact complicated to produce. Here, we show that the most recognizable patterns are characterized not by high feature density but by high spatial dispersion. In this study, our emphasis is on the recognizability of host pattern signatures. Recognizability is subtly different from identifiability in that recognizability refers to the information extracted by the receiver, while identifiability refers to information provided by the signaller [8] . We devised N ATURE P ATTERN M ATCH specifically to investigate recognition of egg patterns from the receiver’s perspective, since ultimately we are interested in whether hosts have evolved eggs that are more recognizable in response to cuckoo mimicry. Are recognizable patterns in fact the most informative and identifiable? Several measures have been proposed to capture the potential information contained in an animal’s signature system, such as Shannon’s information measure ( H s ) [8] . In a future study, it would be productive to compare the available information content of egg patterns (based on objective measures of multiple egg pattern features) to their actual recognizability (as measured here by SIFT-based feature extraction). The idea that hosts of brood parasites might evolve egg signatures originated almost a century ago, when Swynnerton [17] suggested that ‘it is even imaginable that a race may in some cases have taken place between the host’s eggs and those of the overtaking Cuckoo’. Powerful new tools from computer vision studies—a field that is rapidly transforming the study of sensory perception and neurobiology [42] —now make it possible to discover precisely how the race between host and cuckoo eggs has unfolded. Our study provides a first step towards understanding how hosts have evolved individual signatures that are easy to recognize but difficult to forge. As computational neuroscience models become more sophisticated [42] and as we learn more about real-world object recognition in birds [28] , future researchers will be well equipped to investigate not only egg signatures but also broad questions related to recognition (for example, of kin or mates) in other natural contexts. Data collection and digital photography We photographed 689 host eggs from 206 parasitized clutches held in the Natural History Museum (Tring, Hertfordshire, UK). All clutches contained two or more host eggs and 1 (or rarely 2) cuckoo eggs. Clutches belonged to eight principal hosts of the common cuckoo ( Cuculus canorus ) in Europe: dunnock ( Prunella modularis ; n =29; all from England), meadow pipit ( Anthus pratensis ; n =30; all from England), reed warbler ( Acrocephalus scirpaceus ; n =29; all from England), garden warbler ( Sylvia borin ; n =23; 10 from Germany, 7 England, 3 Czech Republic, 2 Pomerania, 1 Poland), great reed warbler ( Acrocephalus arundinaceus ; n =26 clutches; 25 from Hungary, 1 from Germany), brambling ( Fringilla montifringilla ; n =13; 12 from Finland, 1 Russia), pied wagtail ( Motacilla alba ; n =26; all from England) and red-backed shrike ( Lanius collurio ; n =30; 19 from Germany, 6 England, 1 Czech Republic, 1 Poland, 1 Austria, 1 Hungary, 1 Pomerania). To avoid pseudoreplication, we selected clutches from different localities, from different years, or obtained by different collectors. Most eggs were collected between 1880 and 1940. Although egg pigmentation can be susceptible to fading, these effects were minimized because eggs were stored in a dark, controlled environment. Following a protocol described in detail previously [13] , we photographed all eggs using a Fujifilm IS Pro ultraviolet-sensitive digital camera. All images contained a Spectralon grey reflectance standard (Labsphere, Congleton, UK) and were linearized with respect to light intensity [43] . Images were taken at the same distance and angle from eggs. Although colour is an important feature of host eggs, and future studies should assess its contribution to egg signatures, we focused here on egg pattern only. Therefore, we undertook image analysis in terms of a bird’s luminance channel, which is encoded by a bird’s double cones and is believed to be responsible for texture and pattern processing in birds [30] . To convert images to bird luminance, we compared the known spectral sensitivities of the camera [13] with spectral sensitivities of a blue tit’s ( Cyanistes caeruleus ) double cones [44] and transformed the images accordingly. The blue tit’s visual system is believed to be similar to that of other higher passerines [45] . N ATURE P ATTERN M ATCH : a pattern recognition and matching tool We developed a pattern recognition and matching tool, N ATURE P ATTERN M ATCH , using the C++ computer language. The tool uses the Scale-Invariant Feature Transform (SIFT) [26] , [27] , a computer vision algorithm used to detect local features in an image. N ATURE P ATTERN M ATCH operates in two stages: pattern extraction and pattern matching. First, the SIFT algorithm extracts distinctive features from an image. Each feature encodes a normalized gradient orientation histogram in the vicinity of a particular keypoint at a specific scale of analysis, which is chosen by means of a Gaussian scale space representation of the image. Second, we developed a novel pattern-matching algorithm that computes all possible pairwise matchings between populations of features represented in each image. Most approaches to SIFT matching are designed for tasks such as image stitching or object detection, where a particular subset of features representing an object needs to be located in another image [27] . Conversely, N ATURE P ATTERN M ATCH implements an image-to-image pattern matching algorithm that encapsulates the notion of texture similarity as opposed to object identity. Rather than mapping one image to another, the tool considers all possible pairings of individual features from each pair of images. Based on a similarity score calculated for each pair of images, N ATURE P ATTERN M ATCH then ranks the candidate matches in order from most to least similar. On egg patterns, SIFT features are associated with individual blotches and markings ( Fig. 2a ) and represent information on the shape, contrast and dominant orientation of markings. SIFT features are largely invariant to changes in image location, scale and rotation. SIFT features share similar properties with neurons in the primate inferior temporal cortex [26] , [29] and likely correspond to features important for object recognition in other vertebrates, including birds [28] . SIFT has revolutionized computer-assisted recognition tasks in the field of computer vision and has recently been used to recognize handwriting [46] , detect forged digital images [47] and identify individual wild animals based on their markings [48] , [49] . SIFT’s usefulness to evolutionary biologists has so far been restricted to biometric identification [48] , but we believe it can be powerfully implemented in research on animal signalling, recognition and communication as well as pattern formation and development. N ATURE P ATTERN M ATCH was designed with these applications in mind and can be used to recognize and compare natural patterns in a diverse array of animal and plant taxa. N ATURE P ATTERN M ATCH is free and available to the scientific community at naturepatternmatch.org . A comprehensive technical description of N ATURE P ATTERN M ATCH is provided in Supplementary Note 1 . Quantification of signature features To calculate the overall signature recognizability for a given host species, we used N ATURE P ATTERN M ATCH to compare each egg (the reference egg) to all other candidate eggs (a dataset including eggs from its own ‘correct’ clutch and eggs from all ‘incorrect’ clutches). An egg-to-clutch similarity score was calculated based on the average match of the reference egg to all eggs in a clutch, and this score was used to rank the clutches from best to worst match ( Supplementary Fig. 2 ). We calculated the percentage of times an egg’s correct clutch was in the top three matches, a metric that is not overly sensitive (very good matches will still be counted) but sufficiently robust to outliers (poor matches will be excluded). We averaged the ‘top three’ accuracy scores for all eggs to obtain a species-wide grand average and used this as our measure of overall signature recognizability. Our measures of intraclutch and interclutch variation are based on the widely used method of multi-dimensional scaling (MDS). For each species, we first applied our pattern recognition method to compute a distance matrix (where distance=1– similarity score) of all egg-to-egg pairwise similarity distances. Using Matlab’s ‘mdscale’ routine, we then carried out non-metric MDS on that matrix using default parameters to project optimally the data onto two dimensions based on the egg-to-egg similarities. This representation allowed us to employ statistical tools of cluster analysis to assess the degree of variation within and between clutches. In our case, each cluster consisted of the eggs of a particular clutch, as represented by corresponding points within the MDS subspace. Further details can be found in Supplementary Note 1 . For each clutch, we computed the centroid and the distances from that centroid to all eggs in the clutch. Intraclutch variation was quantified as the mean distance between the elements of the clutch and its centroid, averaged over all clutches for a particular species. Interclutch variation was quantified as the mean distance between the centroids of all clutches for a particular species. We also considered related measures of cluster analysis such as the Davies–Bouldin index and the Dunn index. Our measures differ from these slightly in that we required two variables that clearly represent the two different kinds of variation (intraclutch and interclutch) in the data, rather than just a single measure of cluster coherence. Our approach to assessing similarity between eggshell patterns on the basis of SIFT features takes account of the scale and appearance of features but does not explicitly encapsulate their density or spatial arrangements. As a measure of visual complexity, we calculated the average number of SIFT features detected on all eggs for that species, which we subsequently log-transformed to ease direct comparisons. Our measure of visual complexity was insufficient to capture important spatial variation in pattern markings. Although there are several ways to quantify aspects of spatial variation in two-dimensional patterns, we calculated a simple measure of spatial dispersion. For a given species, we calculated the mean distances between all features of any given egg and computed the mean across all eggs belonging to our sample for that species. We also characterized each egg by its mean marking size (based on the average scale of all features), variation in marking size, the percentage of markings in each of four size classes, distribution across marking size classes and variation in spatial dispersion (based on the standard deviation of the mean distances between features). These measures are discussed in detail in Supplementary Note 1 . In the original simulation (presented in the main paper), we used all eggs and all clutches for each host species. There are two potential complications. First, within a species, some clutches had two eggs while others had as many as six, which could affect the a priori likelihood that an egg is correctly matched to its own clutch. We repeated the original simulation using only one randomly selected candidate egg per clutch; this created an effective clutch size of 2 (ref. 16 ). The signature recognizability scores obtained using a clutch size of 2 (computed from 25 repeated trials per species) were highly correlated with those obtained in the original simulation ( R 2 =0.98), indicating that clutch size does not have a large effect on signature recognizability. Second, there were different numbers of clutches for each species. The brambling is rarely parasitized and we were only able to obtain 13 clutches, compared with 30 clutches for red-backed shrike and meadow pipit. We omitted the brambling from the original analyses and the results did not change qualitatively. We also repeated the main simulation using the 13 brambling clutches and 13 randomly selected clutches for all other host species (in 25 repeated trials per species). Although the brambling’s signature recognizability did decline relative to the original simulation, signature recognizability scores in this test were highly correlated with those from the original simulation ( R 2 =0.86). Thus, in the main paper we present the results based on all clutches, but we give less value to the results obtained for brambling. In all statistical analyses, host measures were weighted by number of clutches (see below). Detailed methods are provided in Supplementary Note 1 . Statistical analyses We compared signature recognizability to previously established measures of cuckoo mimicry [13] and host rejection rate of non-mimetic eggs [36] . All statistical analyses were undertaken in IBM SPSS Statistics 21. Using the ‘WLS Weight’ option, we weighted measures obtained for each host species by the number of available clutches. All tests were two-tailed and significance was set at α =0.05. In all analyses we used linear regression models, except in describing the relationships between intraclutch and interclutch variation and between recognizability and visual density. For these we used curve estimation, first weighting cases by number of clutches, to determine that a quadratic model best fit the data. In our analyses, we treated each host species as an independent data point because previous comparative work indicates that evolutionary history has probably not imposed much constraint on the evolution of egg appearance by cuckoo hosts used in this study. The diverse signatures we describe here are consistent with this view. Phylogenetic considerations may be important in future studies that include a wider variety of hosts [7] . How to cite this article : Stoddard, M. C. et al . Pattern recognition algorithm reveals how birds evolve individual egg pattern signatures. Nat. Commun. 5:4117 doi: 10.1038/ncomms5117 (2014).